Migrating deformation in the Central Andes from enhanced orographic rainfall Active shortening in the Central Andes shifted from the western to the eastern margin between 10-7 Ma. Here we propose that this shift was primarily controlled by changes in erosion patterns. The uplift of the Andes blocked easterly winds, resulting in enhanced orographic rainfall on the eastern margin and reduced rainfall on the western margin. Lower erosion rates, associated with the arid conditions, caused the western margin to steepen inhibiting internal deformation and the migration of deformation to the eastern margin where it is active today. River channel profiles on the western margin are indicative of long-term transience from an older tectonic event whereas those on the eastern margin reflect ongoing coupled climatic-tectonic feedback. Both critical wedge theory and local-scale fault friction calculations support this interpretation. This work emphasizes the role that orographic rainfall and erosion can have on the orogen-scale development of mountain belts. The Eastern and Western Escarpments of the Central Andes contrast in both deformation style and climate [1] . The eastern side receives annual rainfall amounts of >3500 mm 2 and experiences active shortening and thrusting [3] , whereas the western side is one of the driest places on Earth and is deformed by long-wavelength warping [2] , [4] . The mechanisms, which acted to create this structure are, however, contested [5] , [6] . The climatic and structural differences are most pronounced in the Central Andes between 10° S and 30° S, which comprise five tectono-geomorphic domains that parallel the mountain range ( Fig. 1a ). The Western Escarpment represents a gently folded ramp connecting the Pacific coast with the volcanic arc of the Western Cordillera. The Altiplano plateau has an elevation of ∼ 4 km ( Fig. 1b ) and extends ca 2000 km in N-S direction and 400 km across strike, linking the Western and Eastern Cordilleras [7] . The Eastern Cordillera can be treated as a bivergent wedge of upper crustal rocks [8] , [9] ( Fig. 1c ). Farther east, the Sub-Andes form an east-vergent fold-and-thrust belt made up of Palaeozoic, Mesozoic and Tertiary units [10] that progressively includes Neogene foreland strata of the Chaco foreland basin [11] . 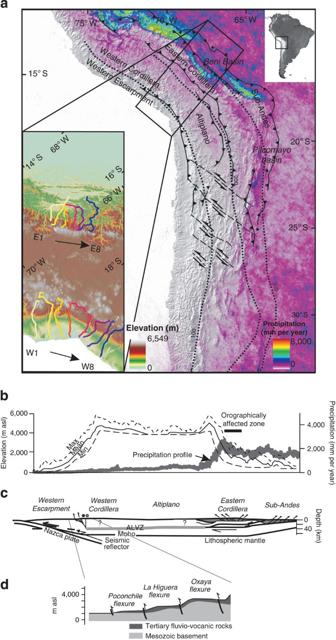Figure 1: Map of the Central Andes and tectonic cross sections. (a) Colour figure illustrating the tectono-geomorphic domains3, the depth of the subducting Nasca plate (dotted lines), the left-lateral faults (dashed lines) dissecting the mountain belt and annual rainfall rates. The inset map shows the streams that were analyzed for this study. Rainfall data are the 2B31 TRMM data set59. (b) A 700 km long topographic cross-section across the Central Andes with maximum, mean and minimum elevations within a 80-km-wide swath extracted from the SRTM 90 m digital elevation model and TRMM rainfall data. (c) Tectonic section showing the architecture on the western margin along with west-ward directed reflectors linking with the ALVZ32, the depth and orientation of the Moho and the ALVZ beneath the Altiplano plateau39, and the tectonic architecture beneath the eastern margin9. (d) Geomorphic details from an 80-km long section of the Western Andean margin showing the surfaces with 6–8° dip angles adjacent to the steeply dipping faults41. Figure 1: Map of the Central Andes and tectonic cross sections. ( a ) Colour figure illustrating the tectono-geomorphic domains [3] , the depth of the subducting Nasca plate (dotted lines), the left-lateral faults (dashed lines) dissecting the mountain belt and annual rainfall rates. The inset map shows the streams that were analyzed for this study. Rainfall data are the 2B31 TRMM data set [59] . ( b ) A 700 km long topographic cross-section across the Central Andes with maximum, mean and minimum elevations within a 80-km-wide swath extracted from the SRTM 90 m digital elevation model and TRMM rainfall data. ( c ) Tectonic section showing the architecture on the western margin along with west-ward directed reflectors linking with the ALVZ [32] , the depth and orientation of the Moho and the ALVZ beneath the Altiplano plateau [39] , and the tectonic architecture beneath the eastern margin [9] . ( d ) Geomorphic details from an 80-km long section of the Western Andean margin showing the surfaces with 6–8° dip angles adjacent to the steeply dipping faults [41] . Full size image Modern moisture is derived from the Atlantic, recycled in the Amazon Basin and transferred to the eastern Andean margin by the low-level Andean jet where orographic effects result in annual rainfall >2000 mm within a ca 20–30 km-wide reach ( Fig. 1b ). Most of this orographic rain falls up to a threshold elevation of 3000 m asl, followed by a decrease to <1000 mm per year towards higher elevations and the Altiplano. The Western Cordillera receives ∼ 200–500 mm per year [5] , [12] , decreasing to nearly zero at the western margin. At large scales structural heterogeneities [5] obscure orogen-parallel trends of positive feedback mechanisms between crustal deformation and the high rainfall gradients [5] . However, climate-driven modulations of rock uplift have been observed for individual domains including the western desert margin [13] and the wet Bolivian Yungas [14] . Here, we link the driest and most humid regions of the Andes perpendicular to strike and propose that the onset of modern orographic precipitation patterns with the rise of the Altiplano ca 7–10 Ma [5] ago inhibited shortening in the west, resulting in tilting and warping of the western margin and in a shift of the locus of shortening to the east where erosion increased [15] . This hypothesis is supported by transient channel morphologies indicative of orographic feedbacks in the east and tectonic-driven knickpoint retreat in the west. Reconstructions of the accretionary wedge geometry on the western Andean margin supports a shift to a super-critical state where deformation only occurs along the basal décollement, whereas on the eastern margin enhanced orographic rainfall promoted thrusting and internal shortening in subcritical to critical conditions. Modelling of high-angle fault movements between the Miocene and today further support an erosion-driven shift in the locus of deformation from the western to the eastern Andes. These findings highlight the strong control that climate and erosion can have on orogen-scale tectonics. Steady state and transient streams Channel profiles are powerful indicators of the long-term forces and short-term perturbations acting on a region [16] , [17] . The timescale of channel response to tectonic and climatic forces depends on uplift and rainfall rates, catchment size and lithology, but is generally estimated to be in the range of 10 6 years for orogen scale rivers [18] . Many channels worldwide are therefore in a transient state, in which a perturbation (climatic or tectonic) has yet to fully propagate through the stream network. The steady state response of a channel to either rock uplift or rainfall variations is identified by a corresponding change in the channel steepness index (provided that the erosivity is constant), whereas the concavity remains constant ( Fig. 2a,b ). However, the transient response of streams to uplift and/or orographic rainfall differs from the steady state solution. For example, an uplift pulse forces streams to adjust by headward retreat, thereby forming a knickzone that separates an upper segment graded to the pre-uplift conditions from a rejuvenated lower reach ( Fig. 2c ). In the knickzone, stream profiles steepen and become more concave to adjust to the lowered base level [18] , [19] . Likewise, orographic rainfall, where a large proportion of the moisture is lost beneath threshold elevations, results in rapid fluvial erosion in the channel reaches with enhanced rainfall. This results in highly concave channel segments where concavity values increase with rainfall gradients [17] , [20] . The presence of highly concave channels implies long-term geomorphic transience as streams return towards lower concavity values at geomorphic steady state [20] . With respect to orogen development, the highly concave nature of orographic rainfall-affected streams results in a reduction in mass compared with lower concavity graded streams [17] , causing an upward compensation of the crust by flexural isostasy [21] , [22] or advection of crustal rocks towards the site of erosion [23] . The flexural response of the crust depends on the magnitude of unloading relative to the flexural rigidity of the lithosphere [21] . The large wavelength of crustal flexural response [22] means that the uplift occurs at much larger spatial scales than the erosional-negative point load [21] , [22] . Crustal advection represents a viable alternative to flexural uplift [23] . This alternative mechanism is a steady-state feedback in which the higher rainfall rates, due to orographic effects, cause enhanced erosion and hence increased rock uplift rates [23] . As in the flexural case, the wavelength of crustal response is large compared with the zone of orographic rainfall-enhanced erosion. The effect is a flattening of the channel gradients upstream and downstream of the high rainfall reach and the development of a broad zone of enhanced channel steepness and concavity ( Fig. 2d ), indicative of high rock uplift and erosion rates at work in the zone of orographic rainfall [16] , [17] , [18] . 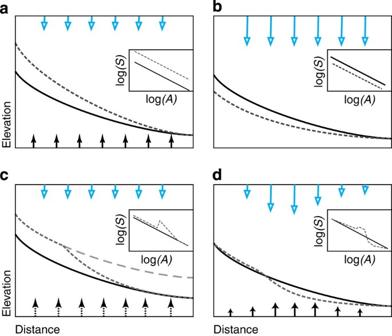Figure 2: Stream responses to tectonic and climate forcing. (a) Steady state response of graded streams to increases in rock uplift rate at constant, uniform rainfall, is a corresponding increase in the channel steepness. (b) Steady state response of graded channels to increases in a uniform rainfall rate at constant rate of rock uplift is a decrease in the channel steepness. (c) A transient response to either a uniform uplift pulse or monoclinal warping results in a transient knickpoint, which moves up the drainage basin16. (d) During active deformation, a positive feedback exists between orographic rainfall and rock uplift with a resulting long-term transient stream profile characterized by a highly concave and steep channels in the orographically affected reach17bordered by relatively flat upper and lower segments24. Open arrows on top: rainfall patterns; closed arrows on bottom: rock uplift patterns. Solid lines: graded stream without perturbation; dashed lines: streams after perturbation. Figure 2: Stream responses to tectonic and climate forcing. ( a ) Steady state response of graded streams to increases in rock uplift rate at constant, uniform rainfall, is a corresponding increase in the channel steepness. ( b ) Steady state response of graded channels to increases in a uniform rainfall rate at constant rate of rock uplift is a decrease in the channel steepness. ( c ) A transient response to either a uniform uplift pulse or monoclinal warping results in a transient knickpoint, which moves up the drainage basin [16] . ( d ) During active deformation, a positive feedback exists between orographic rainfall and rock uplift with a resulting long-term transient stream profile characterized by a highly concave and steep channels in the orographically affected reach [17] bordered by relatively flat upper and lower segments [24] . Open arrows on top: rainfall patterns; closed arrows on bottom: rock uplift patterns. Solid lines: graded stream without perturbation; dashed lines: streams after perturbation. Full size image Streams on eastern margin record crustal response to orographic erosion Streams on the eastern Andean margin are suggestive of long-term transient geomorphic response to climate-tectonic feedbacks. Both the headwater and the lower Sub-Andean reaches exhibit low gradients and low concavities. However, steep and very concave stream segments occur in the zone of enhanced rainfall ( Figs 2d and 3a ), where concavity values increase with rainfall amount ( Fig. 3b,e ), albeit with a weak correlation. However, significant correlations exist with rainfall gradients [24] , as predicted by theory [17] , [20] . Tectonic uplift of rocks can also be inferred in the high rainfall reach based on positive correlations between 10 Be-derived denudation rates and steepnesses of channels [25] . It is not possible to discriminate between geomorphic transience due to flexural accommodation or steady-state crustal advection based on the stream profiles alone. In either case, the maintenance of high concavity values requires flexural accommodation, but it is unlikely that this occurs in the absence of advection as indicated by late Miocene apatite fission track records [26] . 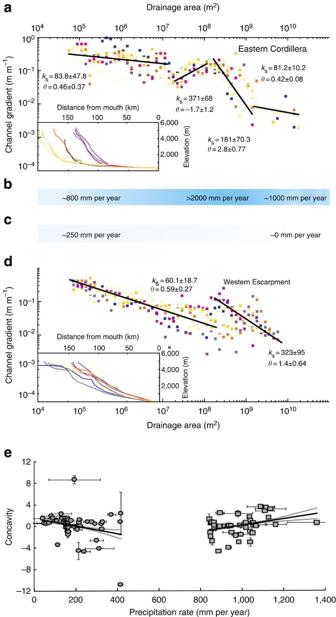Figure 3: Stream geometries of the Central Andes. (a) Log(A)–log(S)diagrams of all analysed streams on the eastern margin. The coloured symbols correspond to the streams fromFigure 1a. (b) Rainfall profiles from the 2B31 TRMM data set59are represented for the eastern margin (darker colours represent more rainfall). (c) Rainfall profiles from the 2B31 TRMM data set59for the western margin (darker colours represent more rainfall). (d) Log(A)–log(S)diagrams of all analysed streams on the western margin. The coloured symbols correspond to the streams fromFigure 1a. (e) The relationships between rainfall rates and concavity values (left: western margin; right: eastern margin) indicate a lack of correlation on the western margin (R2=0.07;P>0.05) and a weak but significant correlation on the eastern margin (R2=0.12;P<0.05). Figure 3: Stream geometries of the Central Andes. ( a ) Log (A)– log (S) diagrams of all analysed streams on the eastern margin. The coloured symbols correspond to the streams from Figure 1a . ( b ) Rainfall profiles from the 2B31 TRMM data set [59] are represented for the eastern margin (darker colours represent more rainfall). ( c ) Rainfall profiles from the 2B31 TRMM data set [59] for the western margin (darker colours represent more rainfall). ( d ) Log (A)– log (S) diagrams of all analysed streams on the western margin. The coloured symbols correspond to the streams from Figure 1a . ( e ) The relationships between rainfall rates and concavity values (left: western margin; right: eastern margin) indicate a lack of correlation on the western margin ( R 2 =0.07; P >0.05) and a weak but significant correlation on the eastern margin ( R 2 =0.12; P <0.05). Full size image Similar river profiles were attributed to the mitigating effects of glacial moraines on stream incision [27] , or glacial erosion in the headwaters [28] . The former is unlikely as orthophotos of the Eastern Cordillera show that end moraines are weakly expressed below ∼ 3500 metres and are, in some cases, situated well above or within the incised valleys [29] , suggesting that channel incision has not been inhibited [24] . We do not exclude glacial erosion, but high 10 Be-derived denudation rates [25] coupled with the highest frequency of landslides in the orographic rainfall-affected reach [30] indicate that fluvial dissection is the dominant process at least over Holocene timescales. In summary, regardless of the role of glaciers in the headwaters and the mechanisms of uplift, the strongly concave high precipitation reach [24] paired with high channel steepnesses [25] requires a positive crustal feedback response to erosion by crustal advection, isostatic compensation or most likely by a combination of both. Streams on western margin record a transient response to rock uplift Streams on the western margin of the Andes commonly exhibit a prominent escarpment with a well-developed knickzone. Upstream of this knickzone, streams have low gradients and curvatures whereas downstream reaches are generally steeper and more concave ( Fig. 3d ). The orbital scale climate variations, which potentially shaped glacial and fluvial segments in the east, are recorded only by cut-and-fill terraces on the western margin [31] . Concavity values do not correlate with rainfall along the entire western margin ( Fig. 3c,e ), indicating a fluvial response to a rock uplift pulse, where a retreating knickzone creates steep channels ( Fig. 2c ). In summary, the channel geometries indicate a fundamental difference between the climatic and tectonic forces at work on the Eastern and Western Andes. Whereas stream morphologies on the eastern side record a positive feedback of rock uplift to orographic rainfall-enhanced erosion, longitudinal stream profiles on the western margin indicate a tectonic driving force only. In the next section, we use mechanical models to explain these differences. Deformation The chronology of tectonic deformation along this transect has been restored based on tectonic and stratigraphic investigations, and low-temperature thermochronometres [3] , [7] , [8] , [9] , [10] , [11] , [26] , [32] , [33] . Although the rate of cumulative shortening across the entire Central Andes has been constant between the Oligocene and the present ( Fig. 4a ), the locus of shortening shifted from the western margin and the Altiplano Plateau to the Sub-Andes between ca 10-7 Ma 3 ( Fig. 4b ). This shift was additionally associated with an acceleration of erosion on the eastern side, as recorded by apatite fission track data [26] and sediment accumulation rates in the adjacent foreland basin [15] . On the western side, the post 10-7 Ma cessation of tectonic shortening [3] was superseded by monoclinal warping [34] . This change was associated with a near-termination of surface erosion on the Western Escarpment as indicated by the preservation of post 10 Ma gravel sheets tens of km [2] in area and fluvial hanging valleys [35] . 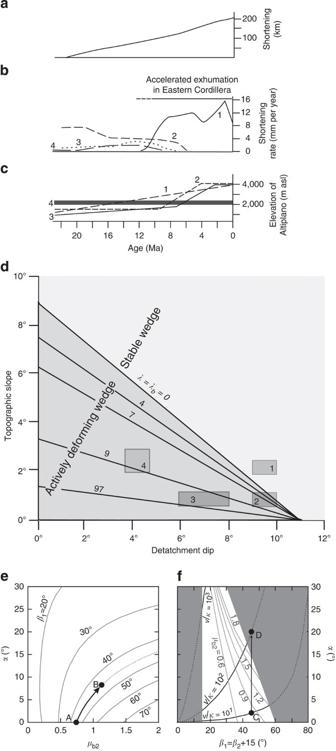Figure 4: Tectonic development of the Central Andes. (a) Cumulative shorting across the entire Central Andes increases steadily3, whereas (b) separate chronologies3show an acceleration of shortening on the east in the Sub-Andes (1) coeval with a reduction in shortening first in the Western Cordillera (4) and Altiplano (3), and finally the Eastern Cordillera (2). (c) Models for the rise of the Andes based on a compilation60proposing a steady rise model (1), structural restorations (2)32,33,41and paleoaltimetry data (3)48. Threshold elevations of 2000–2500 m asl (4) were sufficient to modulate the continental-scale wind and rainfall patterns49,50. (d) Reconstruction of the relationships between topographic slopes and basal décollement angles as a function of fluid pressure ratios whereλandλbdenote the bulk and basal fluid pressure ratios, respectively36, showing the state of the Andes on the desert western margins at the present (1), 20–10 Mya without isostatic considerations (2) and 20–10 Mya including isostatic compensation (3), and on the wet eastern side (4). (e) Deformation model assumingβ1=β2+15°. For the 45° faults on the western margin and 30° faults on the eastern margin, as surface slopes increase from 0° (point A) towards 8° (point B) faults with higher frictional resistance, up toμb2=1.12, will be preferred. (f) A tenfold decrease in erosion shiftsν/κfrom 101(point C) to 102(point D), results in a shift in deformation to structures with order of magnitude higher frictional resistances as the system approaches point D. Point D itself lies in a forbidden zone (grey areas) requiring normal movement on the structures, showing that steady state is unattainable for these parameters. Figure 4: Tectonic development of the Central Andes. ( a ) Cumulative shorting across the entire Central Andes increases steadily [3] , whereas ( b ) separate chronologies [3] show an acceleration of shortening on the east in the Sub-Andes (1) coeval with a reduction in shortening first in the Western Cordillera (4) and Altiplano (3), and finally the Eastern Cordillera (2). ( c ) Models for the rise of the Andes based on a compilation [60] proposing a steady rise model (1), structural restorations (2) [32] , [33] , [41] and paleoaltimetry data (3) [48] . Threshold elevations of 2000–2500 m asl (4) were sufficient to modulate the continental-scale wind and rainfall patterns [49] , [50] . ( d ) Reconstruction of the relationships between topographic slopes and basal décollement angles as a function of fluid pressure ratios where λ and λ b denote the bulk and basal fluid pressure ratios, respectively [36] , showing the state of the Andes on the desert western margins at the present (1), 20–10 Mya without isostatic considerations (2) and 20–10 Mya including isostatic compensation (3), and on the wet eastern side (4). ( e ) Deformation model assuming β 1 = β 2 +15°. For the 45° faults on the western margin and 30° faults on the eastern margin, as surface slopes increase from 0° (point A) towards 8° (point B) faults with higher frictional resistance, up to μ b2 =1.12, will be preferred. ( f ) A tenfold decrease in erosion shifts ν/κ from 10 1 (point C) to 10 2 (point D), results in a shift in deformation to structures with order of magnitude higher frictional resistances as the system approaches point D. Point D itself lies in a forbidden zone (grey areas) requiring normal movement on the structures, showing that steady state is unattainable for these parameters. Full size image We apply two mechanical models to explain the eastward migration of lithospheric shortening. We first apply critical-taper theory [36] , [37] and then assess the role of high-angle faults [38] for shortening the Western and Eastern Cordillera. Deformation as a wedge Mountain belts can be described as orogenic wedges, which reside in either subcritical, critical, or super-critical states depending on the topographic and décollement slopes, and the ratios of the pore water pressure relative to the lithostatic pressure at the décollement and within the wedge [36] , [37] . High basal fluid pressure, indicated by high λ b values on Figure 4d , indicates a mechanically weak décollement horizon, which can sustain a wedge with a low topographic slope. Likewise, high frictional resistance along the décollement, that is, low λ b , will yield a high topographic slope at the state of failure. This critical wedge framework treats mountain belts as an isotropic medium at its plastic limit. Accordingly, deformation occurs internally in subcritical wedges, which are characterized by low surface and décollement angles. Super-critical wedges have steep taper and décollement slopes and deformation is confined to the décollement surface. Critical wedges may deform through both mechanisms [36] , [37] . On the western margin, the latest phase of thrusting occurred between 10-7 Ma and was superseded by long-wavelength warping [34] with the result that the Western Escarpment steepened from ∼ 1° to the current 2–2.5° (refs 32 , 33 ). Pre-7 Ma shortening was accommodated by thrusting along a west-vergent system of steeply dipping reverse faults ( Fig. 1d ) that were kinematically linked with the Altiplano low-S velocity zone (ALVZ) at ca 30 km depth [32] ( Fig. 1c ). Beneath the Altiplano, the top of the ALVZ dips <4° to the west and lies >30 km above the Moho [39] , operating as a shear zone and transferring shortening to the basal décollement beneath the eastern margin ( Fig. 1c ). The décollement horizon is not readily evident in subsurface images of the western margin. However, similar to the situation beneath the Altiplano, it is assumed that the décollement horizon lies within upper crustal units above the Moho, where seismic reflectors dip at 9°–10° to the east and extend from the subducting Nazca plate to the ALVZ ca 60 km farther east [32] ( Fig. 1c ). Accordingly, before ca 10-7 Ma, the 1°-steep topographic slope between the Western Cordillera and the Pacific coast was maintained by a basal décollement horizon 9°–10° steep, or potentially 2°–3° less when considering isostatic adjustments to the lowered topographic loads. The entire wedge at this time resided in the zone of critical to subcritical geometry ( Fig. 4d ), depending on the pore fluid ratios, allowing internal deformation to compensate for changes in crustal accretion and shortening. The modern geometry of the western margin is in a super-critical state ( Fig. 4d ), inhibiting the orogen from further internal deformation [36] , [37] . In this situation, the wedge slides as an intact medium along the décollement where the entire deformation is confined. The current topographic slope on the eastern side is ca 2.2–2.6°, and is maintained by an actively deforming wedge that is detached above the <4° dipping ALVZ [39] ( Fig. 1c ) within the critical to subcritical field ( Fig. 4d ) where internal deformation can occur. Critical/subcritical conditions with lowered topographic slopes and shallower décollements would also have existed in the geologic past. Accordingly, before 7–10 Ma, mass accretion caused deformation of the critical/subcritical frontal segments on both margins. This situation changed after 7 Ma when shortening and related thrusting came to a halt on the super-critical Pacific side and exhumation was accelerated in the Eastern Cordillera [26] , associated with propagation of the deformation into the Sub-Andes [3] . Continued post 7 Ma warping and uplift of the Western Escarpment [34] , as indicated by uplifted Pleistocene marine terraces [40] , does not violate this hypothesis as it need not involve internal deformation. Because the dip angle of the décollement shallows in the up-dip direction ( Fig. 1c ), stable sliding along the décollement results in a passive westward rotation of the entire wedge and in a steeping of the topographic slope. Another likely cause for recent tilting is a change in subduction style. Reduced erosion on the Western Escarpment may have resulted in a change to dry subduction [13] , supporting both steeper subduction and topographic slopes. Therefore, even after the transfer of shortening to the Eastern Cordillera and Sub-Andes, the Western Escarpment could continue long-wavelength warping associated with reduced surface erosion and higher friction on the subducting slab, with stable sliding occurring along the décollement. Deformation and fault friction High-angle faults in both the Western and Eastern Cordillera could invalidate the application of the critical taper wedge model, as it is based on an isotropic medium at its plastic limit. Because of this, we also apply a coupled deformation-erosion model [38] to explore the shift of movement across high-angle faults from a primary to a secondary structure. Hilley et al . [38] showed that erosion, through topography, exerts a major control on the location of deformation where high-angle faults are prevalent. In particular, high topographic slopes increase normal tractions along the primary fault with a friction coefficient, μ b1 . Continued steepening eventually instigates the activation of other higher friction faults, which lack significant topography. We apply mean coefficients appropriate to the Andes that are based on sensitivity studies [38] , and were used to explain fault movements in the Eastern Andes [38] . Reverse faults in the Western Cordillera are from 30°–60° steep ( Fig. 1c ), and surface angles locally reach 8° (ref. 41 ) ( Fig. 1d ), whereas the Eastern Cordillera faults are shallower, averaging 30°, with surface slopes from 2°–4° (ref. 10 ). Based on model results, when surface slopes adjacent to the primary faults grow from 0° (point A in Fig. 4e ) to 8° (point B in Fig. 4e ), the strain would be transferred from the ∼ 45° faults of the Western Escarpment to 30° faults (for example the Eastern Cordillera) with twice the frictional resistance ( μ b1 =0.6 versus μ b2 ∼ 1.1). However, topographic growth and deformation are also tied to erosion. Erosion on the Western and Eastern Escarpment has been quantified over a wide range of time scales. Modern cosmogenic nuclide-derived denudation rates of 0.0001–0.01 mm per year have been measured in northern Chile [42] . Apatite (U-Th)/He exhumation rates in southern Peru from 60-9 Ma [43] are somewhat higher, averaging ∼ 0.01 mm per year. The situation on the Eastern Escarpment differs, with exhumation of 0.2–0.6 mm per year derived from 25-5 Ma apatite fission track ages in the Upper Beni River Basin [44] , and cosmogenic nuclide-derived erosion rates of 0.6–1.3 mm per year during the Holocene [25] . Apatite fission track lengths also imply an acceleration of cooling at ∼ 10 Ma [26] . For the mechanical model used here, the most important observation is that erosion rates on the Western Escarpment are up to 1–2 orders of magnitude slower during the Holocene than before 9 Ma. Likewise, erosion rates on the Eastern Escarpment are 1–2 orders of magnitude faster than on the Western Escarpment, becoming even faster at 10 Ma [26] . Erosion is implemented in the model [38] in the term ν / κ , where ν is the convergence rate and κ is a erosion constant. As with the mechanical model, we assume that the primary (western) structures are at 45° on the average, and the secondary (eastern) structures at 30°. Although κ is not an erosion rate but the erosional efficiency, a tenfold decrease in erosion rate on the Western Escarpment can be modelled by increasing ν / κ from 10 1 (point C in Fig. 4f ) to 10 2 (point D in Fig. 4f ). The resulting increase in the topographic slope above the primary structure would cause migration to secondary structures with order of magnitude higher fault friction, and eventually a shift in the mode of deformation from reverse to normal motion. As predicted by Hilley et al . [38] , in areas of low erosional efficiency such as the Western Andean Escarpment, migration of deformation occurs in preference to topographic steady state. Both models, that is, the wedge and friction fault calculations, support the transfer of shortening from the western to the eastern margin in response to accelerated erosion. The channel morphologies on the western side of the Andes, characterized by a distinct knickzone separating flat headwater segments and steep lower reaches ( Fig. 3d ), reflect the transient response to a rapid pulse of surface uplift ( Fig 2c ), where streams adjusted to the uplift by headward retreat. Low-temperature thermo-chronometry [43] combined with sequential restorations of stream profile geometries [45] suggest that this uplift was accomplished by thrusting along steeply dipping reverse faults [33] ( Fig. 1c ), with internal deformation terminating ca 7 Ma ago [3] . Subsequent warping additionally steepened the streams [34] , [46] , but this mechanism cannot explain the formation of the knickzones as they initiated before 7 Ma [43] , [45] . The channel gradient pattern ( Fig. 3d ) and lack of correlation between concavity values and rainfall rates ( Fig. 3e ) support the kinetic-erosion model results ( Fig. 4f ) that the Western Escarpment has not reached an equilibrium with climate-driven erosion. On the eastern side, the downstream pattern of steepness and concavity values ( Fig. 3a and e ) implies a strong coupling between orographic rainfall-enhanced erosion and tectonic deformation (for example, Fig. 2d ). Accordingly, although the stream morphologies on the western margin record the channel response to a phase of thrusting and shortening that was completed ca 7 Ma ago, the streams on the eastern margin reflect the response of ongoing shortening and related rock uplift modulated by orographic rainfall. This is supported by strain calculations, which show that the Western Cordillera is super-critical whereas the Eastern Cordillera is in a subcritical to critical state. We relate this shift in deformation locus to the rise of the Altiplano above an elevation of ca 2000–2500 m asl, which was the case between ca 14 and 8 Ma ago ( Fig 4c ). This surface elevation rise might have occurred due to the convective removal of the lowermost crust [47] , thermal buoyancy [4] and/or delamination of eclogized lower crust [48] . According to circulation models for moisture transport, these elevations were sufficient to modulate the continental-scale wind and rainfall patterns, and to result in high orographic rainfall gradients in the Eastern Cordillera, enhanced convective rainfall on the Altiplano and the Western Cordillera and blocking of westerly flow from the Pacific [49] , [50] . The consequence was that the arid/hyperarid climate on the Western Escarpment that already persisted before 14-8 Ma [51] became so dry that erosion nearly terminated, as documented by the preservation of post 10 Ma gravel planes and hanging valleys [35] . The deep-seated geodynamic processes above [4] , [47] , [48] could result in an overall tilting of the Western Escarpment leading to the establishment of an orographic rainfall gradient, but cannot be invoked to shift deformation without the dominant effect of rainfall variations, as indicated by channel geometries. The lack of erosion, together with the topographic rise and the steepening of the western ramp, resulted in the triggering of the Lluta collapse, one of largest mass failures on Earth [35] . The steepening of the ramp would have shifted the western margin into a super-critical state and increased the relative friction on steep faults, effectively terminating thrusting on the western side and initiating a period of monoclinal warping. On the eastern margin, the rise of the Altiplano resulted in an acceleration of erosional mass flux since ca 10 Ma [15] through increased orographic rainfall. Higher rainfall rates promoted highly erosive streams, which further enhanced crustal deformation through positive feedback mechanisms, thereby accelerating exhumation in the Eastern Cordillera and promoting active deformation in the Sub-Andes. Our interpretation has implications for the large-scale development of the Andes. Specifically, if orographic rainfall-controlled erosion is responsible for the eastward shift in deformation, then the weakening and eventual reversal of the orographic rainfall pattern towards the south requires a similar reversal in the deformation and exhumation patterns. Our hypothesis predicts the largest changes south of the region from the Beni basin where rainfall rates decrease from >3500 mm per year at 16° S, to the Pilcomayo basin at 20° S with ca 1000 mm per year, as seen by the shift towards low channel concavities and gradients [14] . This is indeed supported by north-south reversal trends of apatite fission track ages [26] , [44] , [52] , [53] , and a series of left-lateral transtensional faults ( Fig. 1a ). These structures dissect the entire crust of the Puna Plateau between 21° S and 28° S and are associated with the ascent of magma [54] , [55] . Slip along these faults has been reactivated through changes in the stress regime [55] , [56] , and particularly in response to a change from dominantly vertical thickening to orogen-parallel stretching [55] . The influence of these faults is strong particularly for the post 7.9 Ma volcanic activities on the plateau, as inferred from age-density analyses of volcanoclastic rocks [54] . As these faults accommodate orogen-parallel variations in shortening [55] and are not related to subduction geometries [55] , we suggest that the reactivation of these faults may also be related to orographic-rainfall induced changes in erosion rates that caused the transfer of shortening from the western margin to the Eastern Escarpment in the Central Andes. Calculation of stream profiles We explore both steady and transient responses to tectonics and climate by a channel's steepness and concavity [16] , [17] . We proceed by using basic relationships between uplift, rainfall, the upstream size of the drainage basin and erosion. At topographic steady state, rock uplift U is compensated by surface erosion E , which depends on the channel bed's shear stress [57] : where k b denotes the erosivity that depends on lithology, climate and sediment load [16] , S channel gradient, Q water discharge, R rainfall rates (assuming no evaporation or infiltration) and A the size of the upstream drainage basin. The gradient of a steady state stream is therefore Channel gradient has also been formulated based on empirical relationships with the basin area [58] : where k s and θ denote channel steepness and concavity indices, respectively. Accordingly, a stream segment can be characterized by k s and θ , whose values are obtained through regression analysis of log (S) versus log (A) . This relationship has the same form as equation (2), where: We use then equation 4 to identify variations in rock uplift and rainfall patterns from channel morphologies. Mechanical calculations We use critical wedge solutions and estimates of surface and décollement angles to estimate the mechanical states on both sides of the Andes [36] , [37] . We then apply the coupled deformation-erosion model of Hilley et al . [38] to calculate the tractions along faults and to explore the shift of slip from a primary to a secondary structure. According to these authors [38] , the friction coefficient of the secondary structure, μ b2 , can be calculated as a function of the friction coefficient of the primary structure, the Hubbert–Rubey pore fluid pressure ratios, λ , for each fault, the topographic slope, α , and the dip angle of the primary and secondary faults, ß 1 and ß 2 . Erosion in the model is based on stream power in which the fluvial erosion coefficients m and n are equal to 0.4 and 1, respectively (equation 1), and the channel width-basin area exponent, h , is 1.6. We applied λ =0 to the primary and secondary faults. We use these median values because they were tested by Hilley et al . [38] for the Andes. How to cite this article: Norton, K. & Schlunegger, F. Migrating deformation in the Central Andes from enhanced orographic rainfall. Nat. Commun. 2:584 doi: 10.1038/ncomms1590 (2011).